Lasing from individual GaAs-AlGaAs core-shell nanowires up to room temperature Semiconductor nanowires are widely considered to be the next frontier in the drive towards ultra-small, highly efficient coherent light sources. While NW lasers in the visible and ultraviolet have been widely demonstrated, the major role of surface and Auger recombination has hindered their development in the near infrared. Here we report infrared lasing up to room temperature from individual core-shell GaAs-AlGaAs nanowires. When subject to pulsed optical excitation, NWs exhibit lasing, characterized by single-mode emission at 10 K with a linewidth <60 GHz. The major role of non-radiative surface recombination is obviated by the presence of an AlGaAs shell around the GaAs-active region. Remarkably low threshold pump power densities down to ~760 W cm − 2 are observed at 10 K, with a characteristic temperature of T 0 =109±12 K and lasing operation up to room temperature. Our results show that, by carefully designing the materials composition profile, high-performance infrared NW lasers can be realised using III/V semiconductors. Semiconductor nanowire (NW) lasers provide the potential to generate highly localized, intense monochromatic optical fields in a geometry that is very well suited to an efficient coupling to highly integrated nanophotonic elements and optical circuits [1] , [2] , [3] , [4] , [5] , [6] , [7] , [8] , [9] . Indeed, the high refractive index of typical semiconductor materials allows the physical size of lasers to be scaled down to only a few hundred nanometres, while the unique NW geometry naturally facilitates low-loss optical waveguiding and optical recirculation in the active region. To date, lasing from NWs has been demonstrated using a range of different material systems that span the ultraviolet and visible regions of the spectrum. This includes ZnO [10] , group-III nitrides [11] , II/VI materials [12] and, most recently, III/V NWs [13] , [14] , [15] , [16] , [17] . Very recently, infrared lasing has been observed at low temperature using InGaAs nanoneedles grown epitaxially directly on silicon [14] and silicon metal oxide semiconductor field-effect transistors [15] by exploiting whispering gallery-like optical modes. Furthermore, first indications of amplified spontaneous emission and lasing have been reported from optically pumped GaSb [16] and GaAs-GaAsP core-shell NWs [17] . For NW lasers that use GaAs as a gain medium, theoretical analyses of the modal gain [13] , [18] , [19] have indicated that continuous wave lasing should be possible in detached NWs. The end-facet reflectivity (~0.6) is sufficient to reach transparency in NWs with a length of a few micrometres by engineering the confinement of the optical mode via their diameter [7] , [13] . However, the deleterious impact of non-radiative surface and Auger recombination has limited progress in the technologically important near-infrared spectral range, although lasing is predicted to be within the reach of GaAs NWs with sufficiently high crystalline quality and lengths exceeding a few micrometres [13] , [20] . In the present work, the NW surface is optically passivated using a thin AlGaAs layer to circumvent the strong non-radiative recombination [21] , [22] caused by the high density of defect states at the GaAs surface. We report room temperature lasing above the amplified spontaneous emission regime with a high T 0 value of 109±12 K and single-mode lasing at 10 K with a remarkably low threshold pump power of 0.76±0.15 kW cm −2 from individual GaAs-AlGaAs core-shell NWs. Sample preparation of GaAs-AlGaAs core-shell NW lasers The GaAs-AlGaAs core-shell NW-laser structures were grown using solid source molecular beam epitaxy (MBE) on a [111] orientated Si substrate (see Methods section). Before growth, the substrates were thermally oxidized and chemically treated to produce a ~2 nm thick SiO 2 mask layer with ~5–10 nm wide pinholes that act as nucleation sites for the self-catalysed MBE growth. Precise control of the axial and radial growth rates of GaAs and AlGaAs was achieved by varying the temperature and III/V flux ratio during MBE growth. Initially, a seed GaAs NW core was synthesized in a self-catalysed (Ga droplet mediated) vapour–liquid–solid growth mode [23] . The NWs thus produced have lengths in the range from 11 to 16 μm and a diameter of 80±5 nm. The need for single-mode transverse optical confinement within the GaAs core and low-loss waveguiding along the NW axis calls for core diameters in excess of ~300 nm ( Supplementary Fig. S1 ). Consequently, the growth conditions in the MBE chamber were adjusted for pure radial GaAs overgrowth (see Methods), until the NW diameter reached 340 nm. Transmission electron microscopy and Raman spectroscopy measurements performed on similar reference samples [24] showed that these growth conditions give rise to NWs with predominant zincblende crystal structure and twin plane defects, that is, unit cell-sized inclusions of wurtzite crystal phase in an otherwise zincblende matrix. To strongly enhance the optical efficiency of the GaAs NWs, the core was overgrown with a 5-nm-thick AlGaAs passivation layer and finally capped with a thin layer of GaAs to prevent oxidation ( Supplementary Fig. S2 ) [25] . 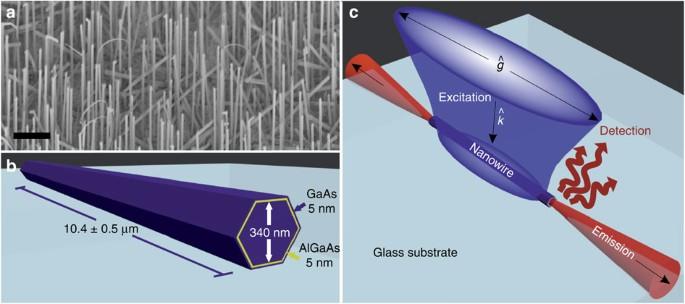Figure 1: As-grown GaAs/AlGaAs NWs and schematic measurement geometry. (a) Scanning electron microscopic image of the as-grown core-shell GaAs-Al0.25Ga0.75As NWs revealing typical lengths ranging from 11 to 16 μm and an areal density of the order of ~108cm−2. Scale bar, 5 μm. (b) Schematic representation of a NW transferred onto a glass microscope slide showing the active GaAs core with a nominal diameter of 340 nm, the 5-nm-thick AlGaAs diffusion barrier and 5 nm thick surface capping layer. (c) Schematic representation of the measurement geometry used for optical measurements in our experiment. The propagation direction of the incident excitation field () is perpendicular to the NW axis and the linearly polarized excitation field is polarized in a direction () parallel to the NW axis to maximize the incoupling efficiency. Emission is detected with a ~0.8 μm spatial resolution along an axis parallel to −. Figure 1a shows a typical scanning electron microscopic image of the as-grown NW-laser structures, with lengths varying from 11 to 16 μm. After growth, the NW lasers were mechanically removed from the growth substrate and spatially dispersed onto a SiO 2 substrate. Figure 1b shows schematically the core-shell NW geometry of such a transferred NW laser, in which the end facets define a longitudinal Fabry–Pérot (FP) laser cavity. Figure 1: As-grown GaAs/AlGaAs NWs and schematic measurement geometry. ( a ) Scanning electron microscopic image of the as-grown core-shell GaAs-Al 0.25 Ga 0.75 As NWs revealing typical lengths ranging from 11 to 16 μm and an areal density of the order of ~10 8 cm −2 . Scale bar, 5 μm. ( b ) Schematic representation of a NW transferred onto a glass microscope slide showing the active GaAs core with a nominal diameter of 340 nm, the 5-nm-thick AlGaAs diffusion barrier and 5 nm thick surface capping layer. ( c ) Schematic representation of the measurement geometry used for optical measurements in our experiment. The propagation direction of the incident excitation field ( ) is perpendicular to the NW axis and the linearly polarized excitation field is polarized in a direction ( ) parallel to the NW axis to maximize the incoupling efficiency. Emission is detected with a ~0.8 μm spatial resolution along an axis parallel to − . Full size image Spectroscopy of GaAs-AlGaAs NW lasers To characterize the optical response of individual NWs, we performed photoluminescence (PL) spectroscopy. As depicted schematically in Fig. 1c , the substrate containing well-dispersed NWs was placed in a He-flow variable temperature cryostat and optically excited with light, linearly polarized along the NW axis. Hereby, a × 100 microscope objective (numerical aperture ~0.6) was used that provides diffraction-limited performance and a minimum spot diameter of ~1 μm. Optical excitation was using a Ti:sapphire laser tuned to 780 nm that provides ~150 fs duration pulses at a repetition frequency of 82 MHz (duty cycle ~10 −5 ). By inserting an f =1 m focal length cylindrical lens into the excitation beam, the excitation channel produces an elliptical focus with a full width at half maximum along the major and minor axes of 5.3±0.2 and 1.6±0.2 μm, respectively ( Fig. 1c ). Emission was also collected along a direction normal to the NW axis and focused into a single-mode optical fibre that provides a detection spot size <1 μm 2 , which can be precisely scanned along the length of the NW. 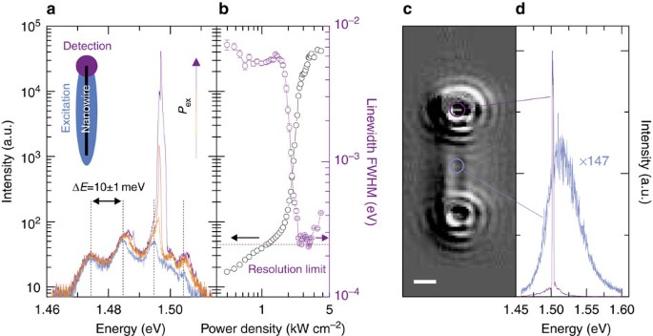Figure 2: Power-dependent and spatially resolved measurements at 10 K. (a) Power-dependent spectra of the scattered light recorded from the end of a single NW as a function of the mean excitation power density. The four curves plotted correspond to excitation power densities of ~1.35, 1.9, 2.4 and 4.8 kW cm−2. Note the logarithmic scaling of the intensity axis and the clear FP modulation of the spontaneous emission, with peaks separated by 10±1 meV denoted by the vertical-dashed lines. The inset shows a schematic depiction of the excitation and detection spots on the NW used to record the spectra. (b) Power dependence of the peak intensity within a ~10 meV wide spectral window centred at 1.495 eV and the linewidth of the dominant emission feature. (c) Image of the NW emission recorded at ~1.5 ×Pthresholdshowing clear interference fringes around the NW end facets and much weaker, spectrally broad spontaneous emission from the body of the NW, extending up to ~1.60 eV. Scale bar, 2 μm. (d) Comparison of the stimulated and spontaneous emission spectra from the NW excited under the same conditions is depicted inc. Input-output characteristics of the NW lasers at 10 K Figure 2a shows a typical series of PL spectra recorded at 10 K from a region close to one end of the NW as the average excitation power density used to excite the entire wire is increased from ~0.4 to 5 kW cm −2 . For the lowest excitation power density, the emission spectrum consists of a relatively broad emission band extending from ~1.46 to 1.51 eV, the dominant emission appearing at ~1.49 eV, below the expected low-temperature zincblende bandgap of GaAs at ~1.515 eV [26] , [26] . The comparatively large bandwidth of the emission spectrum and the observed red shift of the peak emission most probably reflect the presence of twin defects in the GaAs NW core. Such twin defects lead to the formation of indirect excitons with holes confined in the twin plane and electrons in the surrounding zincblende phase [27] , [28] and give rise to an inhomogeneously broadened emission spectrum [29] . In addition, strongly apparent in Fig. 2a is the periodic modulation of the spontaneous emission intensity reflecting regularly spaced longitudinal FP modes separated by 10±1 meV. The spacing of these modes is expected to be δ E =( ħ πc)/( n group · L ), where n group = n eff − λ ( d neff / dλ ) is the group index of the axial guided mode [19] with an effective mode index n eff and L is the NW length (see Methods section). We measured L for all the NW lasers using optical microscopy and calculated the group indices n group =4.85 and 4.86 for the transverse electric (TE) 01 - and transverse magnetic (TM) 01 -guided modes, respectively. Hence, the expected mode spacing between TE/TM-like longitudinal FP modes of NW-A, measured to have a length of 10.2±0.8 μm is 12.5±1 meV, in close agreement with the measurements ( Fig. 2a ). As the excitation laser power density increases beyond ~1.5 kW cm −2 a sudden and highly nonlinear increase in the emission intensity is observed, with a pronounced peak emerging close to ~1.496 eV that rapidly grows to become several orders of magnitude stronger than the background emission. This is clear evidence of population inversion in the NW and amplified spontaneous emission from the end facets. The strongly superlinear increase of the peak emission with pump intensity is consistent with expectations when the laser threshold is approached [30] , [31] . Figure 2: Power-dependent and spatially resolved measurements at 10 K. ( a ) Power-dependent spectra of the scattered light recorded from the end of a single NW as a function of the mean excitation power density. The four curves plotted correspond to excitation power densities of ~1.35, 1.9, 2.4 and 4.8 kW cm −2 . Note the logarithmic scaling of the intensity axis and the clear FP modulation of the spontaneous emission, with peaks separated by 10±1 meV denoted by the vertical-dashed lines. The inset shows a schematic depiction of the excitation and detection spots on the NW used to record the spectra. ( b ) Power dependence of the peak intensity within a ~10 meV wide spectral window centred at 1.495 eV and the linewidth of the dominant emission feature. ( c ) Image of the NW emission recorded at ~1.5 × P threshold showing clear interference fringes around the NW end facets and much weaker, spectrally broad spontaneous emission from the body of the NW, extending up to ~1.60 eV. Scale bar, 2 μm. ( d ) Comparison of the stimulated and spontaneous emission spectra from the NW excited under the same conditions is depicted in c . Full size image The peak intensity of the most intense PL feature is plotted in Fig. 2b as a function of the excitation power density, exhibiting a clear ‘s-like’ dependence that is characteristic of the transition from spontaneous emission to amplified spontaneous emission, and finally to lasing [30] . Far above the threshold, the output from the single mode at 1.496 eV is several orders of magnitude stronger than the spontaneous emission background, and evolves linearly with the pump power density as expected. In previous studies of GaAs/GaAsP core-shell NWs [17] , strong ‘gain-pinning’ effects, indicative of local heating by the excitation laser are evident in the results of ref. 17 where a transition to an output saturation was observed after only a modest (approximately sixfold) enhancement of the emission intensity. In contrast, the results presented in Fig. 2b show that the laser output in our experiments increases by more than three orders of magnitude before a linear lasing regime is established. Furthermore, gain-pinning effects are not evident in our experiments for any of the excitation conditions used. The very clear threshold and strongly nonlinear input-output characteristic is attributed to the high quality of the lattice-matched GaAs/AlGaAs material system [25] in combination with the homogeneous optical excitation of the entire NW. As such, the results presented in Fig. 2 are characteristic of the intrinsic levels of performance that are attainable using GaAs-AlGaAs NW lasers. The linewidth of the predominant luminescence line is also plotted in Fig. 2b . It reduces from ~6 meV for P <1 kW cm −2 to below the resolution limit of our spectrometer (~0.25 meV) for P >1.5 kW cm −2 . The observation of the threshold behaviour, highly nonlinear input-output characteristics and pronounced linewidth narrowing are strong evidence of lasing in the GaAs-AlGaAs core-shell NW, with a threshold power density of P th =2.40±0.45 kW cm −2 for this particular NW. Estimation of the carrier concentration close to threshold Figure 2c shows a charge-coupled device image of the emission of another NW from the same batch with a similar behaviour, pumped above threshold (~1.5 × P th ) at 10 K. As shown in Fig. 2d , the PL spectra recorded from the middle and one end of the NW are entirely different. While very strong and spectrally narrow emission is observed at the NW end facet owing to scattering of laser emission into our detection system, much broader and weaker emission is recorded from the midpoint of the NW. This stems from the weak residual spontaneous emission from the excited NW and provides direct information about the excitation level of the gain material in the lasing regime. The high-energy tail of the spontaneous emission recorded from the NW midpoint extends up to ~1.60 eV, indicative of significant band-filling effects at high excitation levels. To estimate the carrier density close to threshold, we fitted the spontaneous emission spectrum using a simple model, which assumes that the electronic structure of the GaAs core can be described by three-dimensional, isotropic parabolic bands with effective masses =0.063, =0.5 l and =0.08, and that the interband matrix element for optical transitions is constant, independent of energy. Using these approximations, the form of the PL spectrum can be reconstructed by populating the conduction and valence bands, according to their density of states multiplied by the Fermi distribution functions. The excitation level and, thereby, the carrier density controls the relative position of the electron and hole quasi Fermi levels and, therefore, a fit to the emission spectrum provides information on the carrier density and carrier temperature (see Methods section and Supplementary Fig. S3 ). Using this procedure we estimated the electron temperature to be in the range ~130–170 K with a carrier density in the range ~8–12 × 10 17 cm −3 . This range of carrier densities is in good agreement with theoretical predictions of ref. 13 , where threshold gain for similar nanostructures is predicted to be ~200–300 cm −1 for a 10-μm-long NW at ~100 K. This observation further supports our conclusion that we indeed observe lasing from our NW structures. Comparison of optical properties from different NWs We have studied the emission properties of various transferred NWs and found that about 80% of all investigated NWs exhibit the characteristic lasing behaviour described above. 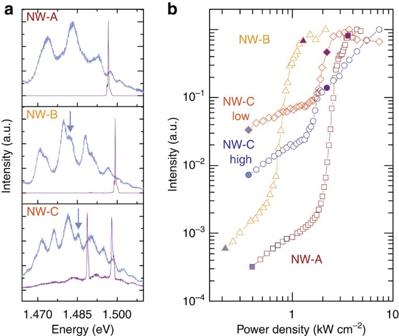Figure 3: Comparison of the lasing performance from different NWs. (a) Output spectra recorded from the end facets of three different NWs with lengths of 10.2±0.8 μm (NW-A), 11.4±0.8 μm (NW-B) and 10.9±0.8 μm (NW-C) with excitation powers below and above threshold, as marked inbby the filled symbols (intensities are normalized). Below threshold, the spontaneous emission is modulated by the FP modes of the cavity. (b) Input-output characteristics of the three NWs as a function of the excitation level, clearly showing the transition to lasing with thresholds at 2.40±0.45 kW cm−2(NW-A), 0.76±0.15 kW cm−2(NW-B) and 1.48±0.3 kW cm−2(NW-C) for the higher-energy lasing peak (NW-C). Figure 3a compares spectra recorded at 10 K from three different NWs, labelled NW-A, -B and -C having lengths of 10.2±0.8, 11.4±0.8 and 10.9±0.8 μm, respectively. For each NW, data are presented in Fig. 3a with excitation power densities below and above threshold, as denoted by the filled blue and violet symbols on Fig. 3b . Below threshold, the emission of each NW exhibits the characteristic periodic modulation that evolves with pump power into single-mode lasing for NW-A and -B and two-mode lasing for NW-C. Below threshold, several longitudinal FP modes are observed in the emission spectrum. For some NWs (for example, NW-A) a single series of longitudinal FP modes is observed, whereas some NWs (for example, NW-B and NW-C) clearly exhibit two series of FP modes, as indicated by arrows in Fig. 3a . This reflects longitudinal modes of two principal transverse-guided modes inside the NW waveguide [13] (TE 01 , TM 01 ) that are calculated to have lowest threshold gain and, furthermore, have a distinct group index (see Methods section). Any reduction of the hexagonal symmetry of the NW, for example, arising from the fluctuating growth environment of specific NWs, shadowing effects and growth competition or, also the shape of the NW end facets, can lift the degeneracy of the TE 01 - and TM 01 -guided modes and both lateral modes compete for gain. The strongest splitting of the FP-mode spectrum is observed in NW-C, which finally results in a bi-modal lasing and clear evidence for modal competition, while NW-A and NW-B exhibit single-mode lasing over the entire range of pump levels investigated. Figure 3b shows the characteristic input-output characteristics of the three NWs as a function of excitation level normalized to the intensities far above threshold. All three NWs clearly show the transition from spontaneous emission to lasing with threshold power densities of 2.40±0.45 (NW-A), 0.76±0.15 (NW-B) and 1.48±0.3 kWcm −2 (NW-C). The variations in threshold power densities are probably due to imperfections of the end facets (mirror losses). NW-B exhibits a remarkably low threshold power density of only 0.76±0.15 kW cm −2 , even lower than theoretical predictions [13] , which demonstrates the high quality of the NW-laser structures fabricated. Figure 3: Comparison of the lasing performance from different NWs. ( a ) Output spectra recorded from the end facets of three different NWs with lengths of 10.2±0.8 μm (NW-A), 11.4±0.8 μm (NW-B) and 10.9±0.8 μm (NW-C) with excitation powers below and above threshold, as marked in b by the filled symbols (intensities are normalized). Below threshold, the spontaneous emission is modulated by the FP modes of the cavity. ( b ) Input-output characteristics of the three NWs as a function of the excitation level, clearly showing the transition to lasing with thresholds at 2.40±0.45 kW cm −2 (NW-A), 0.76±0.15 kW cm −2 (NW-B) and 1.48±0.3 kW cm −2 (NW-C) for the higher-energy lasing peak (NW-C). Full size image Temperature dependence of the input-output characteristics Finally, we investigated the influence of varying the lattice temperature on the NW-laser characteristics. Typical results obtained are presented in Fig. 4a–c from NW-B, which exhibited the lowest threshold power. 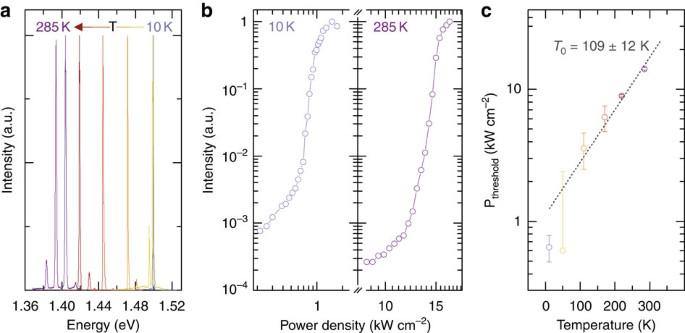Figure 4: Temperature-dependent input-output characteristics. (a) Temperature-dependent emission spectra (normalized intensity) recorded from NW-B pumped above threshold for 10, 50, 110, 170, 220 and 285 K. (b) Input-output characteristics measured at 10 and 285 K from the same NW. (c) Threshold pump power as a function of temperature revealing the characteristic temperature ofT0=109±12 K. The threshold pump power was determined by fitting the output intensity above threshold and extrapolating this curve to thexaxis. The intersection with thexaxis and the corresponding errors that result from the linear fit determines the threshold pump power. Figure 4a,b shows normalized emission spectra recorded above threshold for various temperatures as well as the measured input-output characteristics. Remarkably, clear lasing behaviour is observed up to room temperature. Figure 4a compares normalized spectra recorded above threshold for lattice temperatures ranging from 10 to 285 K. As the lattice temperature varies, the dominant lasing energy red shifts from 1.50 to 1.39 eV, perfectly reflecting the expected bandgap reduction of the GaAs core (see Methods section and Supplementary Fig. S4 ). This observation indicates that the temperature dependence of the NW-laser emission energy is dominated by the bandgap reduction at higher lattice temperatures and that the variation of the refractive index plays a comparatively minor role. Most importantly, since the coefficients extracted from fitting an empirical Varshni dependence to the laser peak energy are very close to expectations for GaAs ( α =5.1±0.8 × 10 −4 eV K −1 and β =84±56 K, c.f . 5.5 eV K −1 and 225 K for GaAs [32] ) while the pump power needed to reach threshold increases exponentially with temperature (see Fig. 4c ), we conclude that heating of the NW lasers via the excitation laser is not significant (see Methods and Supplementary Fig. S4 ). Finally, we note that multimode lasing is observed for temperatures above 220 K, indicative of a temperature-induced reduction of the peak gain [13] and broadening of the gain spectrum to a level comparable to the mode spacing. Laser operation is maintained up to room temperature giving rise to the characteristic input-output curves as shown in Fig. 4b that compares data obtained at 10 and 280 K. The laser threshold power density increases by a factor of ~22 × as the temperature is raised from 10 to 280 K ( Fig. 4c ). This can be fitted by an exponential function describing the thermal broadening of the gain spectrum, and we obtain a remarkably low characteristic temperature of T 0 =109±12 K for this NW laser [33] . Figure 4: Temperature-dependent input-output characteristics. ( a ) Temperature-dependent emission spectra (normalized intensity) recorded from NW-B pumped above threshold for 10, 50, 110, 170, 220 and 285 K. ( b ) Input-output characteristics measured at 10 and 285 K from the same NW. ( c ) Threshold pump power as a function of temperature revealing the characteristic temperature of T 0 =109±12 K. The threshold pump power was determined by fitting the output intensity above threshold and extrapolating this curve to the x axis. The intersection with the x axis and the corresponding errors that result from the linear fit determines the threshold pump power. Full size image We investigated detached GaAs-AlGaAs core-shell NW lasers to characterize and probe their intrinsic properties and performance. Our results showed that the AlGaAs shell inhibits non-radiative surface recombination such that clear near-infrared lasing operation can be achieved up to room temperature in this important materials system. The highly nonlinear input-output emission characteristics have strong potential for novel applications in which lasing is used to optically sense the local environment of the NW [34] or in the use of coupled cavity concepts for switching [35] . Although one can expect further improvements of the NW-laser performance by improving the end-facet reflectivity via chemical polishing or by placing them onto patterned substrates for which distributed feedback concepts can be exploited [36] , the direct integration of III/V NW lasers onto silicon substrates for integrated photonics and optical interconnects [37] remains a significant challenge. Vertical emission has been recently observed from InGaAs-GaAs nanopillars grown on silicon [14] and silicon metal oxide semiconductor field-effect transistors [15] by exploiting low-loss helically propagating modes for which the reflectivity of the NW substrate is high, despite the low index contrast. Furthermore, AlGaAs-GaAs NW lasers could be directly integrated into silicon and III/V photonic crystal nanostructures to facilitate highly directed vertical emission [38] or transferred onto photonic waveguides for use as integrated sources [39] . However, using III/V NWs as an integrated source for applications such as silicon optical interconnects should take advantage of the ability to grow NWs site selectively and, furthermore, the lasers should emit unidirectionally into the underlying silicon photonic hardware. In this context, dielectric Bragg mirrors could be deposited on the as-grown NWs to provide high mirror reflectivity at the upper NW facet and weaker reflectivity at the NW-substrate interface [40] by virtue of the weaker evanescent mode coupling. Such approaches would have significant promise since they may facilitate the realization of compact NW lasers epitaxially on silicon photonic nanostructures, without the need for complex wafer-bonding techniques [41] . For such integrated photonics applications, we note that the emission wavelength must also be shifted further into the infrared, for example, by replacing the GaAs core with InGaAs. Recently, promising first results have been obtained showing that InGaAs NWs with very high uniformity can be grown site selectively on Si and their composition can be tuned over large ranges [42] . This provides significant prospects to extend the emission wavelength into the telecommunications window and beyond for which NW lasing could be obtained providing that Auger losses, which are more significant at longer wavelengths, can be overcome. Finally, electrical injection would be essential for NW lasers operating in an integrated setting. To date, only a few works report lasing from electrically excited NWs [4] , [43] . However, radial p – n junctions in GaAs-based NWs exist driven mostly by potential applications in NW photovoltaics [44] . The availability of such materials provides much promise for the future development of electrically driven, compact III/V NW-laser sources grown site selectively on silicon photonic hardware with the potential for NWs to make a breakthrough in the development of optical interconnects. Growth of core-shell GaAs-AlGaAs NW lasers The GaAs-AlGaAs core-shell NWs were grown using solid source MBE on Si(111) substrates that were thermally oxidized to produce a 20±1-nm-thick SiO 2 mask layer. Before growth, the oxide was thinned using an aqueous, dilute NH 4 -HF solution to produce a ~2-nm-thick SiO 2 layer containing pinholes to the Si(111) substrate, which act as nucleation sites for NW growth [23] , [24] , [45] , [46] . The prepared substrates were then transferred into a Gen II MBE system and held at 700 °C for 20 min to remove surface contaminants before being cooled to the nominal growth temperature of 610 °C. GaAs NWs were synthesized in a self-catalysed (Ga-droplet mediated) vapour–liquid–solid growth mode [23] using Ga and As fluxes of 0.025 and 0.103 nm s −1 , respectively. Growth for 210 min resulted in NWs with a length of 11–16 μm and a core diameter of 80±5 nm. The need for strong optical mode confinement requires NW diameters exceeding 300 nm ( Supplementary Fig. S1 ), which was achieved by a subsequent overgrowth step. For this, the temperature was cooled down to 490 °C while arsenic and gallium fluxes were increased to 0.19 and 0.17 nm s −1 respectively, resulting in a radial growth of GaAs until the desired core diameter of 320 nm is reached. Transmission electron microscopy and Raman spectroscopy measurements performed on reference samples grown under similar conditions [24] showed that the NWs produced have a predominant zincblende crystal structure with occasional twin plane defects in the middle region of the NWs and heavier twin defect densities at the bottom and top ends of the NWs. To strongly enhance the optical efficiency of the NWs and facilitate single-mode optical waveguiding, the GaAs NW core was overgrown with a thin AlGaAs passivation layer and completed with a thin layer of GaAs to prevent oxidation. Hereby, the Al flux was set to 0.057 nm s −1 to grow a 5±1-nm-thick Al 0.25 Ga 0.75 As radial shell around the GaAs core. Finally, the Al cell was closed to grow a 5±1-nm-thick GaAs protection layer on the NW surface. Further details pertaining to the growth procedure of GaAs-AlGaAs core-shell NWs and their structural and morphological properties can be found in refs 24 , 25 . Photonic properties of NW waveguides The as-grown NWs are expected to support optical waveguiding along their axis, characterized by the effective index and mode confinement factor (Г) in the active GaAs region. A commercial-grade simulator (lumerical mode solutions, lumerical finite difference time domain solutions) was used to perform the calculations for the NWs attached to the silicon substrate. The results of these simulations are presented in Supplementary Fig. S1 that shows the calculated optical confinement factor as a function of the NW diameter. Here the NW is placed onto a glass substrate as in the experiments. As shown by Supplementary Fig. S1a , an increase of the NW diameter from 200 to 400 nm is accompanied by a strong increase of Г from ~0.4 to 0.9 as the mode becomes increasingly localized in the active GaAs core of the NW. For the TE 01 mode that propagates in 360 nm core-shell NWs studied in the present manuscript, we calculated an optical confinement factor Г=0.89. The high dispersion of the modes that support lowest threshold gain in a 360-nm diameter core-shell NW [13] leads to a calculated effective refractive group index of n group =4.85 for the TE 01 and n group =4.86 for the TM 01 . Both are indicative of a FP-mode spacing of 10 meV for NWs with L ~11 μm used in this work. The form of the guided optical fundamental mode in the in-plane (axial) direction is also shown in Supplementary Fig. S1b , demonstrating the excellent overlap of the guided mode with the ~360 nm diameter GaAs core, the formation of FP modes in the axial NW resonator and the predominant losses from the end facets. Our finite difference time domain simulations indicate that the maximum reflectivity of the fundamental TE 01 mode at the NW end facets is 58%, translating to a maximum mode Q -factor of the FP resonator modes of Q max ~750, corresponding to a finesse of 5.7 for an 11-μm-long NW. This compares fairly well with the typical observed Q -factors of the FP modes of the spontaneous emission recorded below threshold ( Figs 2 and 3 of manuscript) for NW-A that is measured to be Q =300±150, corresponding to a finesse of 1.9±0.7. Influence of AlGaAs passivation shell on NW core PL yield To determine the vital role of the lattice-matched AlGaAs shell for the NW lasers, we have performed detailed characterizations exploring the influence of the passivation shell on the optical yield from the NW core. Essentially, by employing thin AlGaAs shells carrier diffusion to the NW surface is suppressed [47] , [48] . Our studies indicate that already <10-nm-thick Al 0.3 Ga 0.7 As shell is entirely sufficient to prevent carrier diffusion to the surface and thereby enhance the internal quantum efficiency of the NW core. This fact is clearly demonstrated in Supplementary Fig. S2 showing the relative PL yield from a series of NWs grown under nominally identical growth conditions as a function of the shell thickness in the range of 0–100 nm. These data clearly show that a shell with thickness even as low as 8 nm results in a ~10 3 -fold enhancement in the luminescence efficiency, which dramatically reduces the intrinsic losses of the NW core and makes lasing even up to room temperature possible [25] . Method to estimate the carrier density close to threshold The high-energy tail of the spontaneous emission spectrum shown in Fig. 2d reflects the energetic distributions of electrons in the conduction band and holes in the valence band in the highly excited NW. This is determined by the level of excitation in the NW core (that is, the separation of the electron-μ e and hole-μ h quasi Fermi levels) and the band densities of states (that is, assuming isotropic three-dimensional parabolic bands). Owing to the much lower effective mass of the conduction and heavy hole bands ( m e ~0.068 and m hh ~0.51), the form of the high-energy tail of the PL spectrum is dominated by the form of the electron distribution in the conduction band. Subject to these approximations, it can be shown that the PL intensity as a function of the emission energy ( I ( E ph )) can be written as where is an arbitrary constant and is the bandgap of the GaAs NW. Fitting this expression to the form of the PL spectrum provides us with the position of the electron and hole quasi Fermi levels and the carrier temperature ( ). Supplementary Fig. S3 shows typical results obtained using this procedure. Once the parameters , and T have been obtained, the carrier densities can be extracted using for the electron density and for the holes. The requirement that n = p (charge neutrality) provides and internal consistency check, which is used to check the validity of our approach. Typical results of this procedure provide n = p =0.8–1.2 × 10 18 cm −3 as quoted in our manuscript. Insignificance of heating induced by pump laser Supplementary Fig. S4 shows that the peak positions of the lasing modes as a function of cryostat temperature clearly adhere to expectations from an empirical Varshni fit for GaAs (the rigid red shift observed between the peak positions of the lasing modes and the bulk GaAs data is due to the existence of twin defects, as discussed in the Results and Discussions of the manuscript). Most importantly, since the coefficients extracted from the Varshni fit are very close to expectations for GaAs ( α =5.1±0.8 × 10 −4 eV K −1 and β =84±56 K, c.f . 5.5 eV K −1 and 225 K for GaAs [32] ) while the pump power need to exceed threshold increases exponentially with temperature (see Fig. 4c ), we conclude that laser heating has no crucial influence on the lattice temperature of the NW lasers. We believe that these observations indicate that the cold-finger temperature corresponds very closely to the lattice temperature of the NWs. How to cite this article: Mayer, B. et al. Lasing from individual GaAs-AlGaAs core-shell nanowires up to room temperature. Nat. Commun. 4:2931 doi: 10.1038/ncomms3931 (2013).